Manifestation of unconventional biexciton states in quantum dots Although semiconductor excitons consist of a fermionic subsystem (electron and hole), they carry an integer net spin similar to Cooper-electron-pairs. While the latter cause superconductivity by forming a Bose–Einstein-condensate, excitonic condensation is impeded by, for example, a fast radiative decay of the electron-hole pairs. Here, we investigate the behaviour of two electron-hole pairs in a quantum dot with wurtzite crystal structure evoking a charge carrier separation on the basis of large spontaneous and piezoelectric polarizations, thus reducing carrier overlap and consequently decay probabilities. As a direct consequence, we find a hybrid-biexciton complex with a water molecule-like charge distribution enabling anomalous spin configurations. In contrast to the conventional-biexciton complex with a net spin of s =0, the hybrid-biexciton exhibits s =±3, leading to completely different photoluminescence signatures in addition to drastically enhanced charge carrier-binding energies. Consequently, the biexcitonic cascade via the dark exciton can be enhanced on the rise of temperature as approved by photon cross-correlation measurements. Excitons carry a net spin of either 1 or 2 and are regarded as bosons. Their condensation into one macroscopic wave function [1] , [2] , however, is hampered by a couple of obstacles—to mention two of them, the fermionic substructure impairing the transition temperature [3] , [4] and the frequently fast radiative decay [5] , [6] . The latter can be cured by a spatial separation of the electron and hole subsystem, either using two coupled quantum wells with a superposed electric field [7] , [8] or by a single quantum well with a strong inherent electric field induced by the piezo- and/or pyroelectricity of the crystal lattice [9] , [10] , [11] , [12] . Depending on the size of the vertical charge carrier separation, the excitons exhibit a significant dipole character, thus introducing repulsive dipole–dipole interactions that hinder the formation of multiple exciton complexes. In the case of quantum dots (QDs), the confinement along all three directions in space completely alters this picture. First of all, the confined excitonic complexes are not anymore primarily bound together by Coulomb interaction; their possible dissociation is prevented by the surrounding confinement potential [13] . As a result, a large number of excitonic and charged excitonic complexes can easily form, almost regardless of the binding energies between the component particles [14] , [15] . Only for QDs in the strong confinement regime [16] , [17] , [18] , a biexciton (XX) in its ground state consists of two electrons and two holes occupying the lowest electron and hole orbitals, each with paired spins. The total spin of the resulting XX is s =0 and this boson can decay into one of the two bright exciton (X) states with s =±1 (refs 19 , 20 , 21 ). Consequently, two pairwise cross-linearly polarized, double-peak signatures are characteristic for the decay cascade XX→X→empty QD state [22] , [23] . Such signatures are routinely analysed to support the identification of excitons and biexcitons in micro-photoluminescence (μ-PL) spectroscopy [13] , [24] , [25] . However, for the majority of wurtzite c -plane GaN/AlN QDs [26] , [27] with diameters larger than ≈6 nm, this picture cannot be valid anymore for the following reasons. The strong internal piezo- and pyroelectric fields separate the electron- from the hole-subsystem and cause a very distinct confinement in the growth-direction ( c -axis) for both charge carrier types. Along lateral directions, the electrons are still subject to a strong confinement in contrast to the weakly confined holes, with their large effective hole mass reducing their effective Bohr-radius a * :=( m e / m * ) ε r a 0 (refs 16 , 17 , 18 ) representing a convenient measure for the critical confinement length of orbital formation. Consequently, no significant orbital structure for holes is present anymore in this, so-called hybrid-XX complex, and Coulomb forces (in particular, the hole–hole repulsion and the exchange interaction) become dominant. Hence, laterally separated hole states with parallel spins are energetically more favourable than those exhibiting antiparallel spins as in the case of strong confinement. In this work, we present our theoretical predictions along with experimental evidence for the formation of such a hybrid-XX system with a net spin of s =±3. This specific spin configuration leads to an energetic luminescence transposition between the bright X and hybrid-XX emission, as the strong repulsive dipole–dipole interaction in the hybrid-XX is naturally counterbalanced by the hole–hole exchange interaction and large correlation effects as approved by our accurate multi-particle interaction calculations. The radiative decay sequence of such a hybrid-XX is, due to angular momentum conservation, fundamentally different if compared with the one of conventional biexcitons with s =0. As its intermediate state is one of the dark excitons ( s =±2) instead of the bright excitons ( s =±1), the first decay stage (XX→X) is strongly altered and requires a spin reversal to proceed to the second stage (X→empty QD). Hence, the entire photoluminescence signature of the hybrid-XX reflects its decay via the dark excitons as approved by our temperature-dependent photon cross-correlation analysis and the underlying photoluminescence spectra along with their particular polarization dependence. On the basis of the presented spectroscopic analysis, we can derive all energetic level spacings involved in the hybrid-XX decay cascade in well agreement with our theoretical predictions, yielding a coherent description for this first member in the class of hybrid-quasiparticles. Extreme biexciton binding energies due to separate hole densities As depicted in Fig. 1 , the spatial separation of confined electrons and holes (a) reduces their charge-related, attractive Coulomb interaction (blue) and their spin-related, repulsive exchange interaction (red). For the conventional-XX complex in Fig. 1b , additional repulsive (red)/attractive (blue) Coulomb interactions between the charge carriers exist. Our simulations of the XX reveal a Coulomb repulsion, which overcomes the lateral confinement of the holes, leading to a separated localization of the hole wave functions at the bottom of the QD ( Fig. 1c ). The XX accordingly forms a hybrid system of two electrons sharing one orbital at the top, and two spatially separated holes at the bottom of the QD. In this configuration, the holes can have parallel spins, thus, reducing the energy of the hybrid-XX via the hole–hole exchange interaction (blue). Owing to the reduced hole–hole Coulomb repulsion and the additional attractive hole–hole exchange interaction (compare Fig. 1 ), the total energy of the hybrid-XX is drastically decreased. 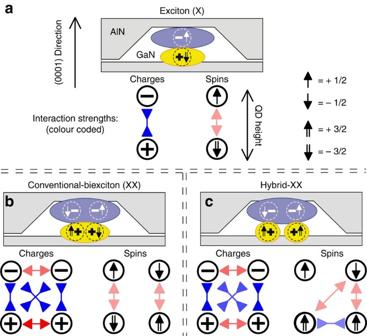Figure 1: Scheme of particle interactions. Schematic arrangement of electron and hole orbitals inside of a wurtzite, c-plane GaN/AlN quantum dot along with their corresponding attractive (blue) and repulsive (red) interactions within the exciton (a) and biexciton (XX) complexes - (b) and (c). Compared with the conventional-XX model (b), a hybrid-XX (c) with a reduced repulsive direct Coulomb and an additional attractive exchange force is energetically more favourable. Figure 1: Scheme of particle interactions. Schematic arrangement of electron and hole orbitals inside of a wurtzite, c-plane GaN/AlN quantum dot along with their corresponding attractive (blue) and repulsive (red) interactions within the exciton ( a ) and biexciton (XX) complexes - ( b ) and ( c ). Compared with the conventional-XX model ( b ), a hybrid-XX ( c ) with a reduced repulsive direct Coulomb and an additional attractive exchange force is energetically more favourable. Full size image A summary of our theoretical and experimental XX-binding energies (X emission energy minus XX emission energy) is given in Fig. 2 . Here, the red circles mark the calculated XX-binding energies for a set of QDs assuming a constant QD aspect ratio ( ar =height/diameter) of 0.2 and a reduced volume with increasing emission energy. Atomic force microscopy and transmission electron microscopy studies confirm such QD aspect ratios between 0.1 and 0.2 (refs 28 , 29 , 30 ) for wurtzite GaN/AlN QDs. Therefore, the assumption of ar =0.2 (red circles in Fig. 2 ) approaches a lower limit for common XX-binding energies, plotted here versus the calculated values of the X emission energies. According to the microscopic analysis, the QDs are modelled as truncated hexagonal pyramids of varying height ( h =0.8–2.4 nm), including a 0.2-nm thick GaN-wetting layer. Our previous results about the excitonic fine-structure splitting [31] show that the QDs have a broken C3v symmetry, here due to an in-plane diameter asymmetry of 20%. Grey dots (metalorganic chemical vapour deposition (MOCVD) growth) and circles (molecular beam epitaxy (MBE) growth [15] ) represent measured XX-binding energies of GaN/AlN QDs in Fig. 2 . Our theoretical results for ar =0.2 nicely match the results for MBE grown QDs and reproduce the sign change of the XX-binding energy, whereas they slightly underestimate the results for MOCVD grown QDs. QD growth kinetics and, thus, the resulting geometries of QDs are known to be different between MBE and MOCVD [32] owing to the fundamentally different growth temperatures. However, the spread of the MOCVD results can be well described by doubling the QD diameter towards ar =0.1, marked by green arrows and the blue line in Fig. 2 , indicating a grid for future explorations. 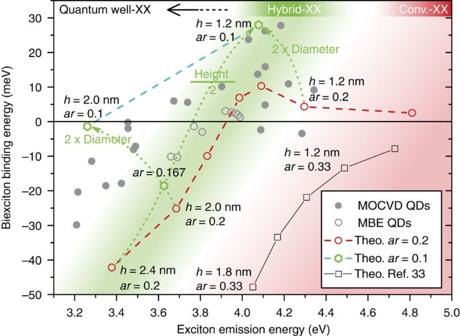Figure 2: Biexciton binding energies. The biexciton (XX)-binding energy (exciton (X) emission energy minus XX emission energy) is plotted versus the X emission energy. Connected red circles show calculated values for quantum dots (QDs) with a constant aspect ratio of 0.2 and reduced height towards larger emission energies. Grey dots depict our experimental data for QDs grown by MOCVD, whereas grey circles show the data for QDs grown by molecular beam epitaxy (MBE) published in ref.15. The experimental results confirm the model of a hybrid-XX not only due to the well-reproduced zero-crossing of the biexciton binding energy, but also due to the modelling of its sheer magnitude. The inclusion of data points for a reduced aspect ratio towards 0.1 (green hexagons and blue line) spans a data grid enclosing the experimental data point spread in well agreement with microscopic studies. Results for the conventional-XX model within another theoretical study33are indicated by black squares for comparison. Figure 2: Biexciton binding energies. The biexciton (XX)-binding energy (exciton (X) emission energy minus XX emission energy) is plotted versus the X emission energy. Connected red circles show calculated values for quantum dots (QDs) with a constant aspect ratio of 0.2 and reduced height towards larger emission energies. Grey dots depict our experimental data for QDs grown by MOCVD, whereas grey circles show the data for QDs grown by molecular beam epitaxy (MBE) published in ref. 15 . The experimental results confirm the model of a hybrid-XX not only due to the well-reproduced zero-crossing of the biexciton binding energy, but also due to the modelling of its sheer magnitude. The inclusion of data points for a reduced aspect ratio towards 0.1 (green hexagons and blue line) spans a data grid enclosing the experimental data point spread in well agreement with microscopic studies. Results for the conventional-XX model within another theoretical study [33] are indicated by black squares for comparison. Full size image Calculations within the conventional-XX model for small QDs with an aspect ratio of 0.33 as shown in ref. 33 ( Fig. 2 , black squares) could not explain the significant zero-crossing of the XX-binding energies [34] , not to mention positive XX-binding energies of up to 30 meV and beyond for even flatter QDs. Our calculations use the same material parameters as refs 33 , 35 , without any artificial reductions of the built-in polarization fields as suggested therein. However, owing to the very large aspect ratios of the model QDs discussed in refs 33 , 35 , all these QDs correspond to the conventional-XX regime of strong confinement. Our non-restricted Hartree–Fock calculations in combination with our experimental evidence predict different biexcitonic regimes, which are marked by coloured areas in Fig. 2 : the conventional-XX (red) for QD diameters ≲ 6 nm, the hybrid-XX (green) with weakly confined holes for QD diameters ≳ 6 nm. For QD diameters ≳ 12 nm, the electrons and holes encounter weak lateral confinement followed by a transition into the quantum-well XX regime without significant lateral confinement. However, please note that the depicted XX-regimes lack well-defined border lines (indicated by colour fading) owing to the wide range of structural QD parameters and are meant for rough orientation only. The orbitals, forming the hybrid-XX, have been calculated by the Hartree–Fock method (see the Simulation Methods subsection and the corresponding isosurfaces of the converged hole densities in Fig. 3b ). The height of the QD can additionally influence this critical diameter, as a smaller electron-hole separation leads to a stronger lateral confinement of the holes by the attraction of the electrons. Prior two-dimensional studies of electron interactions in QDs [36] , [37] , [38] , [39] , [40] raised the question whether a Wigner molecule (of electrons) is reliably described within the unrestricted Hartree–Fock method, allowing for symmetry-broken solutions [41] . Our study uses such a (here three-dimensional) Hartree–Fock method (see the Simulation Methods subsection), which predicts a Wigner molecule-like hole separation within the hybrid-XX model. Therefore, our method might underestimate the minimum QD diameters required for the observed lateral hole separation. However, the agreement between our theoretical and experimental data confirms the entire hybrid-XX model. Although the situation with one strongly and one weakly confined charge carrier type is similar to the situation we found in type II QDs [42] , a (relative to the dark X) negative XX-binding energy would prevent the formation of a XX in such QDs. 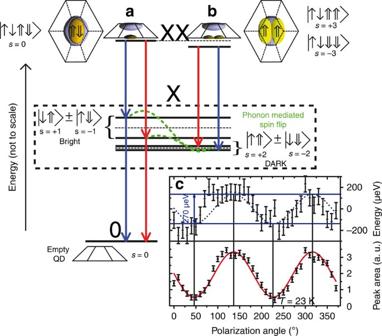Figure 3: Biexcitonic decay cascades. If compared with the conventional-biexciton (XX) (a), the small lateral hole confinement leads to the spatial separation of hole densities in the hybrid-biexciton state (b). The separated holes are allowed to align their spins in parallel, reducing the hybrid-XX energy by the hole–hole exchange interaction. Compared with the conventional-XX (s=0), the hybrid-XX has total spins ofs=±3. Therefore, this complex is able to decay into the dark exciton (X) states withs=±2 via the emission of photons exhibiting an angular momentum of ±1. The energetic splitting of the dark exciton states (μeV) is smaller in regard to the bright X states (meV). An efficient mechanism to depopulate the dark X states is a phonon-mediated spin-flip (green) into the bright X states and the following decay. Polarization-dependent investigations of the XX emission of a quantum dot with a bright X splitting of ≈4.3±0.2 meV (see spectrum inFig. 4a) reveal a small energetic drift of ≈270±50 μeV, representing the dark X splitting (c). Figure 3: Biexcitonic decay cascades. If compared with the conventional-biexciton (XX) ( a ), the small lateral hole confinement leads to the spatial separation of hole densities in the hybrid-biexciton state ( b ). The separated holes are allowed to align their spins in parallel, reducing the hybrid-XX energy by the hole–hole exchange interaction. Compared with the conventional-XX ( s =0), the hybrid-XX has total spins of s =±3. Therefore, this complex is able to decay into the dark exciton (X) states with s =±2 via the emission of photons exhibiting an angular momentum of ±1. The energetic splitting of the dark exciton states (μeV) is smaller in regard to the bright X states (meV). An efficient mechanism to depopulate the dark X states is a phonon-mediated spin-flip (green) into the bright X states and the following decay. Polarization-dependent investigations of the XX emission of a quantum dot with a bright X splitting of ≈4.3±0.2 meV (see spectrum in Fig. 4a ) reveal a small energetic drift of ≈270±50 μeV, representing the dark X splitting ( c ). Full size image Spin properties of confined particles The aligned hole spins of the hybrid-XX cause a total spin of s =±3 (neglecting band-intermixing effects). Therefore, the hybrid-XX can radiatively decay into the dark X states, exhibiting total spins of ±2, comparing Fig. 3a with Fig. 3b . As the electron-hole exchange interaction of symmetry-broken wave functions does not lead to a splitting of the dark X states, in contrast to the bright X states, such dark X states are expected to show a significantly smaller splitting than the bright X states of wurtzite GaN/AlN QDs (with measured bright X fine-structure splittings of 2–7 meV (ref. 31 ); compare the corresponding calculations within Supplementary Fig. 1 (c)). Therefore, the emitted photons of the hybrid-XX show a smaller energetic splitting than expected for a conventional-XX, showing the same splitting as the bright X states [13] , [22] , [23] , [24] , [25] , [43] . Owing to the large total spin of s =±3, μ-PL experiments within magnetic fields should reveal a field strength-dependent fourfold splitting of the hybrid-XX emission line, caused by the splitting of the hybrid-XX states and the dark X states, which will become optically active. Observing such a splitting will be challenging due to the large-emission linewidths [44] but seems achievable based on recent growth advances. However, even without the application of a magnetic field, one can already indirectly witness the anomalous cascade process via the dark states by a straight-forward polarization-dependent μ-PL measurement. A careful analysis of such spectra yields a polarization-dependent shift of the hybrid-XX emission line ( Fig. 3c ) along with a periodic intensity variation, yielding an estimate for the dark X splitting of 270±50 μeV. The corresponding bright X states show a ≈16 times larger splitting of 4.3±0.2 meV as shown in Fig. 4a . A direct comparison between our theoretical and experimental results concerning the polarization of the emission is shown in Fig. 4 for a QD with an emission energy around 4 eV. The depicted contour plots show μ-PL spectra depending on the polarization angle. On top of each contour plot, two single spectra for orthogonal polarization angles are plotted versus the emission energy, demonstrating the fully linear polarization of the bright X states luminescence (X1, X2). The intensities for the corresponding emission lines are plotted versus the polarization angle on the right side of each contour plot for a better identification of the polarization angle-dependent emission maxima. The overlap of two fully cross-polarized XX emission lines in Fig. 4a is mimicking a single, partially polarized emission line [31] . This observation can directly be confirmed by our simulated spectra (b) of the QD structure belonging to the upper green data point in Fig. 2 , which corresponds to an aspect ratio of 0.1 and a biexciton binding energy of ≈28 meV at an emission energy of 4.08 eV. We can observe a striking agreement between experiment and theory that already supports the identification of the hybrid-XX. The only parameters that had to be matched to the experiment for the simulation are the linewidth induced by spectral diffusion [44] , [45] and the particular excitation power and temperature dependencies, varying the intensity balance between X1, X2, XX as shown in Supplementary Figs 2 and 3 . Neither material nor geometric QD parameters were varied to approach the measurement causing the apparent slight discrepancies for the luminescence energies. Therefore, also the bright X states show a QD anisotropy-dependent smaller fine-structure splitting of ≈1 meV in the simulations and a slightly larger hybrid XX-binding energy. The visible emission energy variations of the measured emission lines (a) during the polarization angle scan are caused by the spectral diffusion in GaN/AlN QDs [44] , [45] , which can be suppressed by lowering the temperature, sacrificing the intensity balance of the bright exciton states (see Fig. 5 ). 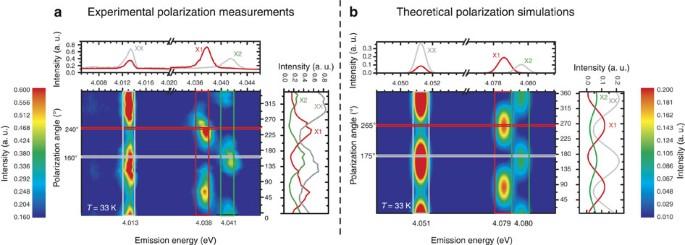Figure 4: Polarization of luminescence. Experimentally recorded (a) and calculated (b), colour-coded polarization spectra are compared with each other yielding a well agreement due to the applied multi-particle calculations. A reduction of the quantum dot aspect ratio towards 0.1 (seeFig. 2) yields biexciton (XX)-binding energies approaching ≈30 meV as reproduced in the comparison shown. The fine-structure splitting between the bright exciton doublets (X1, X2) is influenced by the amount of anisotropy within the quantum dot structure. Figure 4: Polarization of luminescence. Experimentally recorded ( a ) and calculated ( b ), colour-coded polarization spectra are compared with each other yielding a well agreement due to the applied multi-particle calculations. A reduction of the quantum dot aspect ratio towards 0.1 (see Fig. 2 ) yields biexciton (XX)-binding energies approaching ≈30 meV as reproduced in the comparison shown. The fine-structure splitting between the bright exciton doublets (X1, X2) is influenced by the amount of anisotropy within the quantum dot structure. 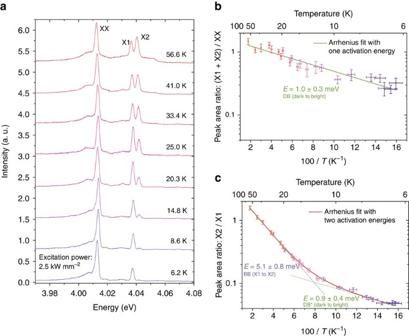Figure 5: Temperature-dependent μ-photoluminescence spectra. Vertically stacked μ-photoluminescence spectra (a) show the bright excitonic (X1, X2) and hybrid-biexciton (XX) emissions depending on temperature. With rising temperature, a thermal activation process strengthens not only X2, but also the overall luminescence intensity of the exciton (X1+X2). The corresponding Arrhenius plots (b) and (c) yield thermal activation energies (EDB(*),EBB), matching the energetic splitting between the dark and bright exciton states. Full size image Figure 5: Temperature-dependent μ-photoluminescence spectra. Vertically stacked μ-photoluminescence spectra ( a ) show the bright excitonic (X1, X2) and hybrid-biexciton (XX) emissions depending on temperature. With rising temperature, a thermal activation process strengthens not only X2, but also the overall luminescence intensity of the exciton (X1+X2). The corresponding Arrhenius plots ( b ) and ( c ) yield thermal activation energies ( E DB(*) , E BB ), matching the energetic splitting between the dark and bright exciton states. Full size image Thermal occupation of exciton spin states Temperature-dependent μ-PL measurements ( Fig. 5 ) reveal the thermal activation of the bright exciton states (X1, X2) due to phonon-mediated spin-flip processes [46] , transferring the carriers between the dark and the bright exciton states. By comparing the overall exciton intensity with its biexciton counterpart in an Arrhenius plot ( Fig. 5b ), one determines an activation energy ( E DB ) of 1.0±0.3 meV resembling the average excitonic dark–bright splitting. Interestingly, the sole thermal activation of X2 in regard to X1 is a two-step process as shown in Fig. 5c . On the basis of a simple Arrhenius fit [47] , we extract two activation energies: E DB* =0.9±0.4 meV, again matching the average excitonic dark–bright splitting; and E BB =5.1±0.8 meV, implying the much larger fine-structure splitting of the bright exciton states. Therefore, both Arrhenius plots independently deduce E DB , in line with the theoretical prediction of an average dark–bright splitting of 0.81 meV, strongly scaling with the QD volume as demonstrated in Supplementary Fig. 1 . The thermal activation of the excitonic emission lines evidences the existence of efficient phonon-mediated spin-flip processes [46] within GaN/AlN QDs. This explains the stronger X1 in comparison with X2 emission in Fig. 4 , despite a much larger oscillator strength of X2 depending on the amount of fine-structure splitting between X1 and X2 (ref. 31 ). In addition, this unbalance in the oscillator strengths explains the observations of E DB* in the low-temperature regime of Fig. 5c . The dark X states as the final states of the initial hybrid-XX decay are expected to be long-time stable until additional carriers are captured by the QD or a phonon-mediated spin flip to a bright X state takes place as illustrated in Fig. 3b . The latter process must be efficient to explain the occurrence of intense X emission besides the hybrid-XX emission. Excitonic spin-flip times of QDs in the order of ps have already been reported [48] and acoustic phonon coupling to excitons in GaN/AlN QDs is exceptionally strong [49] , [50] . The most direct and suggestive proof for the occurrence of phonon-mediated spin-flip processes arises from temperature-dependent second-order correlation functions. At a temperature of 30 K ( Fig. 6a ), one observes the typical signature of a cascade process arising from the decay of the hybrid XX (start) to the ground state via the dark and bright X states (stop). By lowering the temperature to 8 K ( Fig. 6b ), one can efficiently suppress the phonon-mediated spin-flip processes, yielding the typical cross-correlation signature of a XX cascade via an additional intermediate level [51] governing the decay dynamics. Here, the hybrid-XX decay rate ( R 1) is enhanced in comparison with the exciton decay rate ( R 2*), which is limited by the spin-flip rate from the dark into the bright states. Details regarding the convoluted fitting routine [30] , [52] , [53] , [54] can be found in the Supplementary Note 2 . Identical excitation conditions at 30K equalize R 1 and R 2*, proving the existence of a phonon-limited hybrid-XX cascade including a transition from the dark to the bright X states. The apparent temporally broad (≈±25 ns) bunching phenomenon in both correlation functions arises from spectral diffusion [44] , [45] and is modelled as described by Sallen et al . [55] . Further standard techniques for the identification of QD emission lines are discussed in Supplementary Note 2 . Consequently, a phonon-limited hybrid XX→dark X→bright X→empty QD emission cascade is witnessed at low temperatures, which is activated on the rise of temperature. 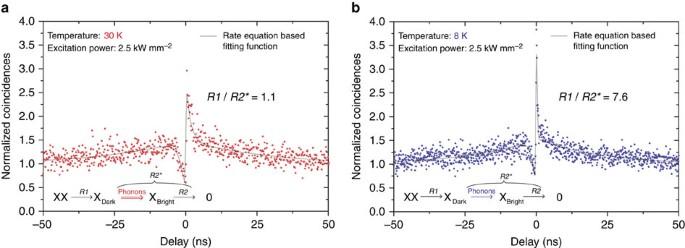Figure 6: Temperature-dependent second-order correlation. Both histograms show the photon cross-correlation analysis comprising the hybrid-biexciton (start) and both bright exciton complexes (stop). By lowering the temperature from 30 K (a) to 8 K (b) at a constant excitation power, one observes the transition from a typical biexciton cascade (a) towards the signature of a spin-blockaded biexciton cascade (b). The weighting between the corresponding ratesR1 andR2* obtained from a fitting procedure (solid line, compared withSupplementary Note 2) is correspondingly altered, clearly demonstrating the influence of the phonon-mediated dark to bright exciton transitions. Figure 6: Temperature-dependent second-order correlation. Both histograms show the photon cross-correlation analysis comprising the hybrid-biexciton (start) and both bright exciton complexes (stop). By lowering the temperature from 30 K ( a ) to 8 K ( b ) at a constant excitation power, one observes the transition from a typical biexciton cascade ( a ) towards the signature of a spin-blockaded biexciton cascade ( b ). The weighting between the corresponding rates R 1 and R 2* obtained from a fitting procedure (solid line, compared with Supplementary Note 2 ) is correspondingly altered, clearly demonstrating the influence of the phonon-mediated dark to bright exciton transitions. Full size image In some of the single-QD spectra, we found additional emission lines that we tentatively assign to charged excitonic complexes by comparison with our artificial polarization spectra (see Supplementary Fig. 4 ). A positively charged X (+X) is expected to show the same spatial hole separation as the hybrid XX. Therefore, all hole and electron spins are expected to align parallel to each other, due to the exchange interaction. The two possible +X ground states with total spins of s =±1/2±3/2±3/2=±3.5 are degenerate and exhibit a high resistance against spin dephasing, which makes the +X in GaN/AlN QDs extremely interesting for quantum-computing applications. The preparation and reading of the +X spin states should be possible in future polarized photon absorption and emission experiments. Experimental details The wurtzite GaN QDs grow by means of low-pressure metal-organic vapour deposition at a density of ≈6 × 10 9 cm −2 . A detailed description of the growth conditions can be found elsewhere [44] , [53] , [56] , [57] . The sample's mesa structures (200 nm–2 μm diameter) were processed by means of e-beam lithography and plasma etching to enable single-QD spectroscopy. We used a frequency-quadrupled solid-state laser emitting at 266 nm as excitation source for the μ-PL spectra. For the temperature-dependent μ-PL measurements, the sample was situated in a Helium flow cryostat and its luminescence was dispersed by a single monochromator equipped with a charge-coupled device array. The optical resolution of this system is better than 200 μeV at a photon energy of 4 eV. A super-achromatic λ/2-waveplate in combination with a linear polarizer (contrast better than 1:5000) was used for measuring the polarization-dependent μ-PL spectra at a constant integration time of 60 s and an angular resolution of 10°. All spectra were calibrated with a mercury gas discharge lamp. For the second-order correlation measurements, the light was guided towards a non-polarizing beam splitter before each light beam was dispersed by an individual monochromator, exhibiting a variable bandpass (optical resolution better than 1meV at a photon energy of 4 eV). The light was finally detected by bialkali photomultiplier tubes with a measured biphoton time resolution of 225 ps. Conventional photon counting electronics were used to obtain the final histograms. Simulation methods The calculation is based on the 8-band-kp formalism described in ref. 58 including the influences of strain, pyroelectricity and piezoelectricity as well as spin orbit and crystal-field splitting. The material parameters from refs 59 , 60 have been included as described in ref. 61 . The sign of one of the piezoelectric constants has been corrected as described in ref. 33 based on the discussions in refs 62 , 63 , see summarizing Supplementary Table 1 . For the calculation of the multi-particle interaction energies, the configuration interaction (CI) method is applied. This method is in principle an exact computation method, yielding the true multi-particle energies, if the number of basis states reaches infinity. Smaller basis sizes produce approximated energies for the respective excitonic complex. Besides the number of states (here we use 10 electron and 20 hole states), the quality of the approximation is sensitive to the quality of the basis states. Instead of single-particle basis states, which were used in a previous 8-band-kp study of GaN/AlN QDs [33] , [35] , we use Hartree–Fock states, representing the best possible basis states for a CI calculation. Hartree–Fock states fully include renormalization effects of particle wave functions by calculating the mean Coulomb and exchange interaction potentials iteratively. Therefore, our CI calculations only need to treat additional correlation effects, enabling us to differentiate between the contributions of renormalization and correlation effects to the particle interaction energies (see Supplementary Note 1 ). By including all interactions of the confined particles, our results are as exact as an 8-band-kp approach can be. As we additionally use realistic geometries for our model QDs, our simulations well describe the experimental observations. How to cite this article : Hönig, G. et al . Manifestation of unconventional biexciton states in quantum dots. Nat. Commun. 5:5721 doi: 10.1038/ncomms6721 (2014).